Carbene organic catalytic planar enantioselective macrolactonization Macrolactones exhibit distinct conformational and configurational properties and are widely found in natural products, medicines, and agrochemicals. Up to now, the major effort for macrolactonization is directed toward identifying suitable carboxylic acid/alcohol coupling reagents to address the challenges associated with macrocyclization, wherein the stereochemistry of products is usually controlled by the substrate’s inherent chirality. It remains largely unexplored in using catalysts to govern both macrolactone formation and stereochemical control. Here, we disclose a non-enzymatic organocatalytic approach to construct macrolactones bearing chiral planes from achiral substrates. Our strategy utilizes N-heterocyclic carbene (NHC) as a potent acylation catalyst that simultaneously mediates the macrocyclization and controls planar chirality during the catalytic process. Macrolactones varying in ring sizes from sixteen to twenty members are obtained with good-to-excellent yields and enantiomeric ratios. Our study shall open new avenues in accessing macrolactones with various stereogenic elements and ring structures by using readily available small-molecule catalysts. Macrolactones, cyclic carboxylic esters with over twelve-membered rings, are broadly present in natural and synthetic functional molecules [1] . Representative examples of bioactive macrolactones include medicinally important macrolide antibiotics such as erythromycin, and agrochemicals like avermectin and Spinosad (Fig. 1A ) [2] , [3] , [4] . The unique conformational (and configurational) properties posed by the macrocyclic structures are critical for these molecules to display the right bioactivities [5] , [6] . Therefore, the preparation of macrolactones has received significant attention over the past decades [1] , [7] , and new synthetic methods continue to emerge in recent years [8] , [9] . One class of such methods starts from substrates with carboxylic ester moieties pre-installed on the main chains and uses various transformations (such as those based on transition metal-catalyzed bond formations) to close the respective macrocycles [10] , [11] , [12] , [13] . The other type of methods, primarily a classic strategy, relies on the formation of carboxylic esters from the corresponding carboxylic acids and alcohols as the ring-closing step (Fig. 1B ) [14] , [15] , [16] , [17] , [18] . Indeed, this lactonization method still constitutes as the most prevalent, reliable approach, and holds clear promise especially since the selective acyl transfer reactions have been well explored through activation of acyl donors by both small-molecule [19] , [20] , [21] , [22] , [23] and enzyme catalysts [24] , [25] , [26] . In the past, studies on macrolactonization mainly focused on developing new carboxylic acid/alcohol coupling reagents and methods to ensure the lactone formations, in which the stereochemical course is mostly controlled by the inherent pre-existing chirality of substrates. There are fewer studies on using catalysts to simultaneously govern the lactonization reaction and stereochemical controls. In 2020, Collins and co-workers showed that the reaction between di-carboxylic acids (tethered with aliphatic linkers) and ortho -substituted benzylic diols can be mediated by the Candida antarctica lipase B (CALB) enzyme catalyst to form macrolactones (Fig. 1C ) [27] . Due to rotational constraints posed by the macrocycles, the macrolactone products feature planar chirality and are obtained with excellent enantioselectivities under the control of the CALB enzyme catalyst. Additionally, it is noteworthy that chiral frameworks with planar stereogenicity are not only of high interest in their distinct molecular chirality, but also broadly present in natural products and utilized in asymmetric catalysis and materials (Fig. 1A ) [28] , [29] , [30] . Despite this elegant work [27] , examples to address the long-standing challenge of catalytic approach toward planar chiral cyclophane molecules remains largely unexplored [31] , [32] , [33] , [34] , [35] , [36] , [37] , [38] . Fig. 1: Importance of macrolactones and the enantioselective synthesis. A Examples containing macrolactone motif and representative planar chiral macrocycles; B Typical synthetic strategy via macrolactonization; C Preparation of planar chiral macrolactones by enzyme catalysis; D Our proposed carbene organocatalytic strategy for planar enantioselective macrolactonization. Full size image We are interested in exploring N-heterocyclic carbene (NHC) as a small-molecule catalyst to address synthetic challenges in complex molecules [39] . NHC is, in principle, a class of excellent acylation catalysts that can offer multiple handles to modulate reactivity and chemo/regio/stereo-selectivities [40] , [41] , [42] , [43] , [44] , [45] . In this work, we disclose a non-enzymatic organocatalytic strategy for efficient access to planar chiral macrolactones (Fig. 1D ). The reaction of the NHC catalyst with aldehyde moiety of the bifunctional hydroxyl aldehyde substrate 1 under oxidative conditions effectively leads to an NHC-bound acyl azolium intermediate [46] , [47] , [48] , [49] . This intermediate then reacts with the alcohol moiety of the substrate to close the lactone ring. The pro-chiral arene planes from substrate 1 in the intermediate are well differentiated by stereo-control of the chiral NHC catalyst, leading to the planar chiral macrolactones 2 with good yields and excellent enantiomeric ratios. In the long round, our study shall open new avenues in accessing macrolactones with various chirality styles and ring structures by using readily available small-molecule catalysts. We commenced our investigation with the expeditious preparation of acyclic substrate 1a (Fig. 2 ). Substituted naphthol aldehyde 4a was easily accessed through a reaction sequence involving a formylation and bromination process from commercially available 1-naphthol ( 3a ). A side chain was subsequently installed with 5a via a Mitsunobu reaction, leading to the desired model substrate 1a through mild deprotection of the TBS group upon treatment with TBAF. Fig. 2: Synthetic protocol of substrate 1a. (1) Titanium tetrachloride, dichloro(methoxy)methane, THF, 0 °C to rt, 10 min; 82% yield; (2) Diisopropylamine, NBS, CH 2 Cl 2 , 45 °C, 16 h; 62% yield; (3) DIAD, PPh 3 , 5a , THF, 0 °C to rt, 12 h; 82% yield; (4) TBAF, THF, rt, 12 h; 60% yield. NBS N -bromosuccinimide, TBS tert -butyldimethylsilyl, TBAF tetrabutylammonium fluoride, DIAD diisopropyl azodicarboxylate. Full size image With the acyclic aldehyde 1a in hand, we set out to study the carbene-catalyzed enantioselective macrocyclization (Fig. 3 ). Gratifyingly, the reaction enabled by achiral NHC A with K 2 CO 3 in toluene at 100 °C gave rise to the desired product 2a in 35% yield, revealing the feasibility of NHC-catalyzed macrolactonization transformation. Various chiral carbene catalysts B - H were then carefully screened to explore their capability for stereo-control over planar stereogenicity of the macrocyclic product 2a . Whereas indanol-based catalyst D afforded the product in modest enantioselectivity (entries 2–4), we were pleased to find that N-2,4,6-trichlorophenyl substituted NHC E was superior to give the product 2a in a promising 75:25 enantioselectivity (entry 5). Further introduction of substituents (e.g. Br and NO 2 ) on the indanol aromatic ring significantly improved the planar enantioselectivity, in which catalyst G furnished the product in 91:9 selectivity, albeit in a modest yield resulting from the competing intermolecular lactonization process to form the dimerization side product (see Supplementary Information for details) (entry 7). 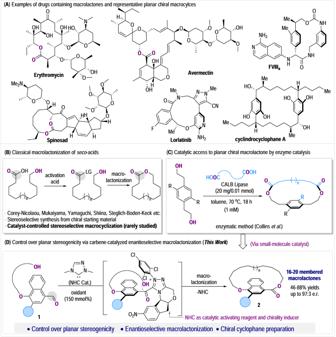Fig. 1: Importance of macrolactones and the enantioselective synthesis. AExamples containing macrolactone motif and representative planar chiral macrocycles;BTypical synthetic strategy via macrolactonization;CPreparation of planar chiral macrolactones by enzyme catalysis;DOur proposed carbene organocatalytic strategy for planar enantioselective macrolactonization. By evaluation of other catalysts, bases (entries 8–11) as well as various solvents and temperatures (see Supplementary Table 1 , Supplementary Information for details), we were delighted to achieve the stereoselective synthesis of planar chiral product 2a with 64% yield and 93:7 er by employment of catalyst G with DABCO as the base (entry 11). Encouraged by the successful examples on cooperative NHC and co-catalysts [50] , [51] , [52] , [53] , [54] , [55] , we then turned to examine various hydrogen bond donors (HBD), as well as Lewis acids/Brønsted acids to further enhance the catalytic performance (Supplementary Table 1 , Supplementary Information for details). Satisfyingly, an optimal condition was obtained utilizing a cinchona-derived HBD- 3 as a cocatalyst in the presence of a mixed solvent (toluene: n -heptane), furnishing the product 2a in 80% isolated yield and 96:4 er (entry 15). The improved results might arise from the additional hydrogen-bonding interaction provided by the thiourea moiety of HBD- 3 with the hydroxyl group and NHC-bound acyl azolium intermediate [31] , [32] , [33] , [34] , [35] , [36] . Furthermore, the use of enantiomeric NHC G ( ent - G ) as the carbene catalyst afforded the product 2a in 70% yield and a reversed 6:94 er (entry 16), indicating a slight match/mismatch relationship between NHC G and co-catalyst HBD- 3 . It is also worth noting that the cyclophane product 2a showed a remarkable configurational stability upon thermal racemization experiment of macrolactone 2a in mesitylene, in which erosion of enantioselectivity was not observed even at 150 °C when the title compound 2a started to decompose. Fig. 3: Optimization of the carbene-catalyzed enantioselective macrocyclization. a The reactions were performed with 1a (6.3 mg, 0.015 mmol, 1.0 equiv. ), NHC A - H (20 mol%), DQ (9.2 mg, 150 mol%), and base (20 mol%) in toluene (1 mM) under N 2 atmosphere at 100 °C for 12 h; b Yields of 2a were determined via 1 H NMR analysis with 1,3,5-trimethoxybenzene as an internal standard; Isolated yield in the parenthesis; c 15 mol% of additive was used; d A mixed solvent (toluene: n -heptane = 11:9, 1 mM) was used. DIEA N, N -diisopropylethylamine, DABCO triethylenediamine, DQ 3,3’,5,5’-tetra-tert-butyldiphenoquinone, HBD hydrogen bond donor. Full size image With the optimal reaction conditions established, we set out to study the generality of the carbene-catalyzed synthesis of planar chiral macrolactones (Fig. 4 ). An array of substituents on the aromatic moiety of aldehyde substrate 1 were initially explored in the catalytic stereoselective macrocyclization. In addition to bromo group, substrates with chloro- and iodo-functional units were readily converted smoothly under the optimal conditions, delivering to the corresponding products 2b and 2c in 61–75% yields with high enantioselectivities (95:5 and 97:3 er, respectively). Installment of a diverse set of aromatic substitutions on the naphthalene moiety of 1 was subsequently studied. To our delight, the 3-phenyl substituted substrate afforded the macrolactone 2d with 81% yield and 93:7 er. 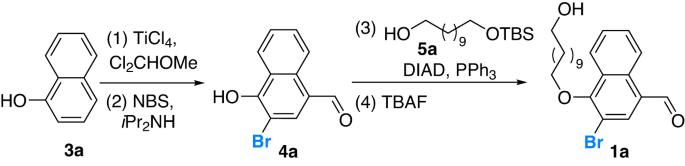Fig. 2: Synthetic protocol of substrate 1a. (1) Titanium tetrachloride, dichloro(methoxy)methane, THF, 0 °C to rt, 10 min; 82% yield; (2) Diisopropylamine, NBS, CH2Cl2, 45 °C, 16 h; 62% yield; (3) DIAD, PPh3,5a, THF, 0 °C to rt, 12 h; 82% yield; (4) TBAF, THF, rt, 12 h; 60% yield. NBSN-bromosuccinimide, TBStert-butyldimethylsilyl, TBAF tetrabutylammonium fluoride, DIAD diisopropyl azodicarboxylate. Various substituents such as Cl, CH 3 , OCH 3 at the para -position of 3-phenyl group showed excellent compatibility under this condition, providing products 2e – g with even higher yields (82–88%) and good stereoselectivities. Furthermore, the 3-aryl unit on the naphthalene core of 1 could be replaced with 2-naphthyl ( 2 h ) and various heteroaromatic units such as thienyl ( 2i ), furyl ( 2j ), benzothienyl ( 2k ) and benzofuranyl ( 2 l ) substituents, which significantly expanded the scope of planar chiral macrolactone derivatives. Further modification of the 3-substituent to 2-position of the naphthalene scaffold with a simple methyl group furnished the product 2 m in 78% yield and 95:5 er. Noteworthy is that [18]-paracyclophanes 2n and 2o with ortho -disubstituted phenyl ring could also be prepared with our method, wherein the NO 2 group was compatible under the catalytic conditions albeit in a slightly dropped enantioselectivity ( 2o , 90:10 er). Notably, these planar chiral products exhibit substantial configurational stability as well, as demonstrated by product 2o , which did not show decreased er value upon heating in mesitylene at 150 °C, while the title compound 2o gradually decomposed. Fig. 4: Substrate scope of the enantioselective macrolactonization. a The reactions were conducted with 1 (0.05 mmol, 1.0 equiv. ), NHC G (5.2 mg, 20 mol%), DQ (30.6 mg, 150 mol%), HBD- 3 (5.2 mg, 15 mol%), and DABCO (1.12 mg, 20 mol%) in toluene/ n -heptane (11:9 v/v, 1 mM) under N 2 atmosphere at 100 °C for 12 h; Isolated yields; b Reactions at 70 °C for 12 h. Full size image Next, we turned to examine the length of the ansa chain to prepare paracyclophanes with various ring sizes (Fig. 5 ). Substrates with a 13-, or 12-membered ansa chain were readily converted to the corresponding planar chiral macrolactones 2p (with a 17-membered macrocycle) and 2q (with a 16-membered macrocycle) in excellent enantioselectivity. Notably, the absolute configuration of the planar chiral macrolactone products was established as ( R p ) [56] by analogy to product 2p via X-ray crystallographic analysis. However, further reducing the ansa chain to 11 members failed to give the corresponding product 2r under the optimal conditions, most likely due to the unfavorable formation of a rigidified macrocycle. On the other hand, the side chain could be readily extended to 15 and 16 members, which produced the products 2s and 2t in 93:7 and 86:14 er, respectively. Furthermore, various functionalized linkers in the ansa chain, such as thioether ( 2u ), 1,3-diyne ( 2v ) and ether ( 2w ), were compatible to deliver the corresponding products 2u – w in modest yields and high enantioselectivities. Fig. 5: Exploration of the ansa chains. a The reactions were conducted with 1 (0.05 mmol, 1.0 equiv. ), NHC G (5.2 mg, 20 mol%), DQ (30.6 mg, 150 mol%), HBD- 3 (5.2 mg, 15 mol%), and DABCO (1.12 mg, 20 mol%) in toluene/ n -heptane (11:9 v/v, 1 mM) under N 2 atmosphere at 100 °C for 12 h; Isolated yields. Full size image The optically enriched planar chiral macrolactones prepared in our approach could readily undergo further synthetic transformations (Fig. 6 ). A palladium-catalyzed Suzuki cross coupling reaction between 2a and 6 afforded chiral cyclophane 7 with 80% yield and 94:6 er. Other transition-metal-catalyzed couplings were also viable to diversify the catalytically obtained macrolactone products. For instance, a Heck reaction with styrene 8 enabled by Pd(OAc) 2 /PPh 3 afforded the alkene-tethered planar chiral macrocycle 9 in 42% yield and 95:5 er. Additionally, Sonogashira coupling of 2c with terminal alkyne 10 led to product 11 in 92% yield and without erosion of er value. Fig. 6: Synthetic transformations of the obtained products 2a and 2c. Detailed reaction conditions for the transformations are presented in the Supplementary Information . Full size image In summary, we have developed a carbene organocatalytic approach for planar enantioselective macrolactonization. 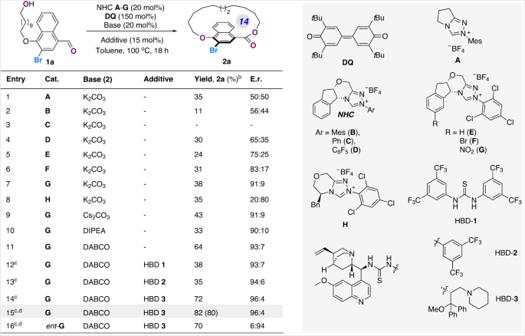Fig. 3: Optimization of the carbene-catalyzed enantioselective macrocyclization. aThe reactions were performed with1a(6.3 mg, 0.015 mmol, 1.0 equiv.), NHCA-H(20 mol%), DQ (9.2 mg, 150 mol%), and base (20 mol%) in toluene (1 mM) under N2atmosphere at 100 °C for 12 h;bYields of2awere determined via1H NMR analysis with 1,3,5-trimethoxybenzene as an internal standard; Isolated yield in the parenthesis;c15 mol% of additive was used;dA mixed solvent (toluene:n-heptane = 11:9, 1 mM) was used. DIEAN, N-diisopropylethylamine, DABCO triethylenediamine, DQ 3,3’,5,5’-tetra-tert-butyldiphenoquinone, HBD hydrogen bond donor. A wide range of cyclophanes, featuring intriguing configurationally stable planar stereogenicity owing to the restricted ring flip of the macrocycles, were obtained efficiently in high yields and excellent stereoselectivities under oxidative NHC conditions. Diversification of the chiral macrocycles were readily achieved through a series of coupling reactions to significantly expand the scope of this method. 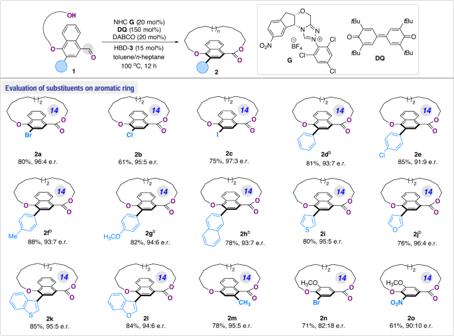Fig. 4: Substrate scope of the enantioselective macrolactonization. aThe reactions were conducted with1(0.05 mmol, 1.0 equiv.), NHCG(5.2 mg, 20 mol%), DQ (30.6 mg, 150 mol%), HBD-3(5.2 mg, 15 mol%), and DABCO (1.12 mg, 20 mol%) in toluene/n-heptane (11:9 v/v, 1 mM) under N2atmosphere at 100 °C for 12 h; Isolated yields;bReactions at 70 °C for 12 h. Furthermore, our approach provides a (non-enzymatic) organocatalytic approach to address the long-standing challenge in stereoselective preparation of planar chiral macrolactones. New avenues by carbene organocatalytic approach for synthetic implementation to access optically enriched planar chiral frameworks and biologically intriguing macrocyclic scaffolds could be anticipated. Ongoing studies in our laboratory include development of the prepared planar chiral macrolactones for chiral catalyst design, and biological activity evaluation for novel agrochemical discovery. To a 100.0 mL Schlenk flask equipped with a magnetic stir bar was added chiral NHC pre-catalyst G (5.2 mg, 20 mol%), DQ (30.6 mg, 150 mol%,), DABCO (1.12 mg, 20 mol%), HBD- 3 (5.17 mg, 15 mol%) and aldehyde substrate 1 (0.05 mmol, 1.0 equiv.). After that, a mixed solvent of toluene / n -heptane (11:9 v / v , 1 mM) was added and the reaction mixture was allowed to stir for 12 h at 100 °C. Then the mixture was concentrated under reduced pressure. 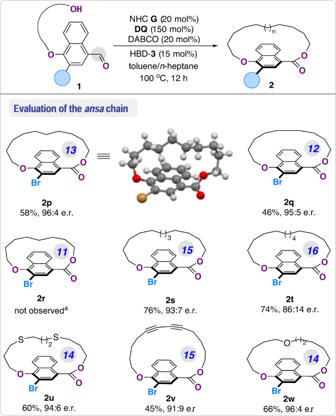Fig. 5: Exploration of theansachains. aThe reactions were conducted with1(0.05 mmol, 1.0 equiv.), NHCG(5.2 mg, 20 mol%), DQ (30.6 mg, 150 mol%), HBD-3(5.2 mg, 15 mol%), and DABCO (1.12 mg, 20 mol%) in toluene/n-heptane (11:9 v/v, 1 mM) under N2atmosphere at 100 °C for 12 h; Isolated yields. 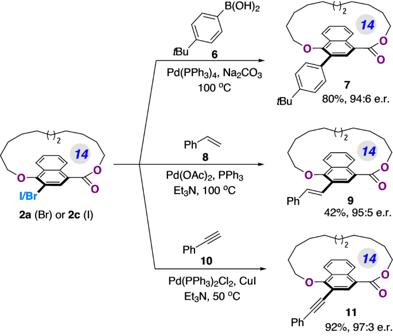Fig. 6: Synthetic transformations of the obtained products 2a and 2c. Detailed reaction conditions for the transformations are presented in theSupplementary Information. The resulting crude residue was purified by column chromatography on silica gel to afford the desired planar chiral product 2 .